An epigenetic switch induced by Shh signalling regulates gene activation during development and medulloblastoma growth The Sonic hedgehog (Shh) signalling pathway plays important roles during development and in cancer. Here we report a Shh-induced epigenetic switch that cooperates with Gli to control transcription outcomes. Before induction, poised Shh target genes are marked by a bivalent chromatin domain containing a repressive histone H3K27me3 mark and an active H3K4me3 mark. Shh activation induces a local switch of epigenetic cofactors from the H3K27 methyltransferase polycomb repressive complex 2 (PRC2) to an H3K27me3 demethylase Jmjd3/Kdm6b-centred coactivator complex. We also find that non-enzymatic activities of Jmjd3 are important and that Jmjd3 recruits the Set1/MLL H3K4 methyltransferase complexes in a Shh-dependent manner to resolve the bivalent domain. In vivo , changes of the bivalent domain accompanied Shh-activated cerebellar progenitor proliferation. Overall, our results reveal a regulatory mechanism that underlies the activation of Shh target genes and provides insight into the causes of various diseases and cancers exhibiting altered Shh signalling. Sonic hedgehog (Shh) signalling, mediated by Patched and Smoothened, functions as a morphogen or a mitogen during many developmental processes [1] , [2] , [3] . Mutations in the Shh pathway components lead to developmental diseases and cancers [4] , [5] . Shh signalling produces specific transcriptional outcomes by differentially regulating the activities of Gli family transcription factors [1] , [2] . Under basal conditions, Gli3, and to a lesser extent Gli2, is processed to generate a truncated Gli repressor (GliR) that represses basal expression of Shh target genes. Shh signalling de-represses and activates target genes by inhibiting Gli3 processing, inducing Gli3 degradation and activating Gli2/Gli1 transcription activators (GliA). The morphogen activity of Shh (for example, in neural tube patterning) is largely dependent on its role as an antagonist of GliR function. GliA-mediated transcription activation in response to Shh is critical for neural tube progenitor specification in the most ventral areas [6] , [7] . The mitogenic effects of Shh in many normal and cancer cell types also require the GliA activities [1] , [2] . For example, Shh/GliA signalling plays a predominant role in the proliferation of early postnatal cerebellum granule neuron precursors (CGNPs) [8] , [9] , [10] , [11] . Mutations that result in constitutively active Shh signalling cause CGNP overproliferation and are the leading genetic causes of the childhood brain tumour medulloblastoma [4] , [5] . Recent studies suggest a link between active Shh pathways and other cancers, and it appears that the oncogenic functions of the Shh pathway require GliA-mediated transcription activation [1] , [4] . Despite extensive studies of Hedgehog signalling in multiple organisms, one fundamental question remains to be answered: how do Gli proteins de-repress and activate target gene expression in response to Shh? Epigenetic factors play critical roles in determining transcription outcomes by regulating chromatin structures and accessibilities of DNA to transcription machineries. Recently, we identified a Brg1-containing chromatin remodelling complex that represses basal expression and activates Shh signalling-induced target gene expression [12] . Interestingly, our results suggest that Brg1 mainly functions as a docking site for other chromatin regulators. Brg1 deletion leads to changes in histone modifications in the regulatory regions of Shh target genes. Thus, additional histone modifiers may regulate Shh signalling, and it is likely that Shh signalling-induced transcription factor exchange from GliR to GliA is accompanied by changes of associated epigenetic cofactor complexes to produce specific chromatin environments and transcription outcomes. Bivalent chromatin domains containing both a repressive H3K27me3 and an active H3K4me3 mark are found in the regulatory regions of many developmental genes in stem cells; these bivalent domains keep gene expression repressed but poised for induction [13] , [14] , [15] , [16] . During development, the resolution of the bivalent domain accompanies the activation or silencing of the poised genes. The PRC2 complex catalyses the addition of H3K27me3 ref. 17 , whereas the H3K27me3-specific demethylases UTX/Kdm6a and Jmjd3/Kdm6b remove it [18] , [19] , [20] , [21] , [22] . UTX is also a subunit of H3K4 methyltransferase MLL2/3 complexes [20] , [23] , which may coordinately activate bivalent genes by removing H3K27me3 and increasing levels of H3K4me3. The Jmjd3 catalytic domain shares homology with UTX; however, genetic analyses indicate that they play distinct roles during development [24] , [25] , [26] , [27] . Although Jmjd3 does not appear to be a subunit of Set1/MLL complexes, it is able to interact with Set1/MLL complexes [21] . The interaction is not strong, and it is not clear whether this interaction plays a role in resolving bivalent domains during bivalent gene activation. How bivalent domains are regulated coordinately by epigenetic factors in response to specific developing signals has not been well understood. In this study, we identified a bivalent domain at the regulatory regions of poised Shh target genes. Shh signalling induces an epigenetic switch to resolve bivalent domains and activates gene expression. PRC2 complexes repress Shh target genes by maintaining the repressive H3K27me3 levels, whereas Shh-induced recruitment of Jmjd3 activates target genes by displacing PRC2, enzymatically removing H3K27me3 and recruiting Set1/MLL complex. The central role of Jmjd3 in regulating Shh-activated gene expression was demonstrated in vivo in Shh activation-dependent development and medulloblastoma growth. Our study reveals an important epigenetic mechanism underlying the gene activation in response to Shh and identifies a potential target to disrupt the mitogenic effect of Shh signalling during tumour progression. Poised Shh-responsive genes are marked by a bivalent domain To understand the chromatin environment of poised Shh target genes, we analysed the publicly available histone modification data obtained from Shh-responsive mouse embryonic fibroblast (MEF) cells (Geo data sets GSE21271 (ref. 28 )). MEFs as well as NIH3T3 mouse fibroblasts express both Gli repressors and activators and are widely used in studies of Shh signalling [29] . Several universal Gli target genes, such as Gli1 , Ptch1 and Hhip , are relatively restricted to the Shh pathway, and their expression reflects Shh/Gli signalling activities. In this screen, we identified an H3K27me3/H3K4me3 bivalent domain in the regulatory regions of these Shh target genes ( Fig. 1a ). The H3K27me3 marks are close to the previously identified Gli-binding regions [30] , [31] . These regions are close to the promoters and may represent proximal enhancers. In contrast, the Shh-independent Gli3 gene was only marked with H3K4me3, whereas a silenced neural-specific target gene Olig2 was only marked with H3K27me3 ( Fig. 1a ). We performed an RNA-seq analysis to compare expression profiles in wild-type MEFs cultured with or without Shh; expression of 25 genes was significantly induced by Shh treatment ( P <0.05). 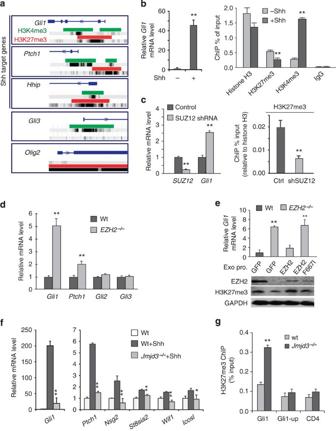Figure 1: PRC2 and Jmjd3 regulate Shh target gene expression by modulating the bivalent domains. (a) Analyses of ChIP-seq data (Geo datasets GSE21271) showed bivalent domains close to transcription start sites of Shh target genes in MEFs. Red and green bars represent the chromatin regions enriched for H3K27me3 and H3K4me3, respectively. The 5′ regions of the genes are shown as blue lines.Gli3is not a Shh target gene;Olig2is a neural-specific Shh target gene not expressed in MEFs. (b) Activation ofGli1by addition of Shh to MEF cultures was associated with decreased H3K27me3 and increased H3K4me3 levels in theGli1regulatory region. The mRNA levels were measured by RT–qPCR, and the ChIP results were analysed by ChIP-qPCR. Histone H3 and IgG ChIP were used as histone and antibody controls, respectively (means±s.d.,n=3). (c) Reducing SUZ12 levels in MEFs by shRNA treatment led to decreased local H3K27me3 levels and increasedGli1expression as shown by RT–qPCR. Histone H3 ChIP was used for ChIP normalization (means±s.d.,n=3). (d) Deletion ofEZH2led to increased basal expression ofGli1andPtch1, but notGli2/3, as shown by RT–qPCR (means±s.d.,n=3). (e) Upper panel: exogenous wild-type EZH2, but not the F667I mutant, rescuedGli1expression defects inEZH2−/−MEFs as analysed by RT–qPCR. Lower panel: western blots show the expression of EZH2 and global H3K27me3 in wild-type andEZH2−/−MEFs (means±s.d.,n=3). (f) Wild-type andJmjd3−/−MEFs were treated with Shh. RT–qPCR analyses ofGli1,Ptch1and other Shh-responsive genes are shown (means±s.d.,n=3). (g)Jmjd3deletion led to higher H3K27me3 levels in theGli1regulatory region in Shh-treated MEFs as shown by ChIP-qPCR. A region upstream ofGli1and theCD4gene were negative controls. Significance was determined usingt-test or ANOVA withpost hoc t-test (means±s.d.,n=3). ** indicatesP<0.01 and * indicatesP<0.05. Eighteen of these contain the bivalent chromatin domain ( Supplementary Table 1 ). Other typical repressive marks, such as H3K9me3 and the PRC1-mediated ubiquitinated H2AK119 (refs 32 , 33 ), were not present. Thus, the poised Shh target genes may be specifically marked by the bivalent chromatin domain. Figure 1: PRC2 and Jmjd3 regulate Shh target gene expression by modulating the bivalent domains. ( a ) Analyses of ChIP-seq data (Geo datasets GSE21271) showed bivalent domains close to transcription start sites of Shh target genes in MEFs. Red and green bars represent the chromatin regions enriched for H3K27me3 and H3K4me3, respectively. The 5′ regions of the genes are shown as blue lines. Gli3 is not a Shh target gene; Olig2 is a neural-specific Shh target gene not expressed in MEFs. ( b ) Activation of Gli1 by addition of Shh to MEF cultures was associated with decreased H3K27me3 and increased H3K4me3 levels in the Gli1 regulatory region. The mRNA levels were measured by RT–qPCR, and the ChIP results were analysed by ChIP-qPCR. Histone H3 and IgG ChIP were used as histone and antibody controls, respectively (means±s.d., n =3). ( c ) Reducing SUZ12 levels in MEFs by shRNA treatment led to decreased local H3K27me3 levels and increased Gli1 expression as shown by RT–qPCR. Histone H3 ChIP was used for ChIP normalization (means±s.d., n =3). ( d ) Deletion of EZH2 led to increased basal expression of Gli1 and Ptch1 , but not Gli2/3 , as shown by RT–qPCR (means±s.d., n =3). ( e ) Upper panel: exogenous wild-type EZH2, but not the F667I mutant, rescued Gli1 expression defects in EZH2 −/− MEFs as analysed by RT–qPCR. Lower panel: western blots show the expression of EZH2 and global H3K27me3 in wild-type and EZH2 −/− MEFs (means±s.d., n =3). ( f ) Wild-type and Jmjd3 −/− MEFs were treated with Shh. RT–qPCR analyses of Gli1 , Ptch1 and other Shh-responsive genes are shown (means±s.d., n =3). ( g ) Jmjd3 deletion led to higher H3K27me3 levels in the Gli1 regulatory region in Shh-treated MEFs as shown by ChIP-qPCR. A region upstream of Gli1 and the CD4 gene were negative controls. Significance was determined using t -test or ANOVA with post hoc t -test (means±s.d., n =3). ** indicates P <0.01 and * indicates P <0.05. Full size image Using Gli1 as a representative Shh target gene, we examined whether the marks in the bivalent domain changed with Shh induction. Using chromatin immunoprecipitation (ChIP), we found that H3K27me3 was present in the regulatory region of Gli1 gene, and levels were significantly reduced on Shh treatment ( Fig. 1b ). H3K4me3 levels in the Gli1 promoter were significantly increased in Shh-treated MEFs ( Fig. 1b ). Similar changes were observed when Gli1 and other Shh target genes were de-repressed in Gli3 −/− MEFs or further activated in Shh-treated Gli3 −/− MEFs ( Supplementary Figs 1 and 2 ). Thus, Gli-mediated Shh target gene de-repression and activation are accompanied with the removal of H3K27me3 and increase in levels of H3K4me3. PRC2 and Jmjd3 are important for Shh target gene expression To determine whether H3K27me3 reduction is a causal factor in the Shh-mediated gene activation, we manipulated the enzymes that add or erase H3K27me3 marks. The PRC2 complex, which methylates H3K27, contains three essential subunits, EZH2, SUZ12 and EED [13] . RNAi inhibition of SUZ12 expression led to decreased local H3K27me3 levels and increased Gli1 basal expression ( Fig. 1c ). In EZH2 −/− MEFs [34] , [35] , global H3K27me3 levels were decreased and basal expression of Shh target genes such as Gli1 and Ptch1 was increased compared with those in wild-type cells ( Fig. 1d ). Neither Gli2 nor Gli3 expression was affected and Olig2 was not de-repressed by EZH2 deletion ( Fig. 1d ). Only the wild type but not an enzymatically inactive mutant EZH2 (F667I) [35] rescued the Gli1 expression defect ( Fig. 1e ). These experiments suggest that the PRC2 complex represses basal Shh target gene expression by maintaining the H3K27me3 mark. This mechanism also provides a possible explanation for the recent findings that EZH2 deletion leads to a de-repression of Shh target genes in developing limbs and dorsal hindbrains [36] , [37] . In MEFs lacking Jmjd3 ref. 25 , an H3K27me3 demethylase, we observed defects in Shh-induced gene activation. The activation of several bivalent Shh-responsive genes identified in RNA-seq experiments ( Supplementary Table 1 ) was significantly impaired in Jmjd3 −/− MEFs ( Fig. 1f ). Jmjd3 deletion resulted in higher local H3K27me3 levels in the Gli1 gene in the presence of Shh ( Fig. 1g ) but not in higher global H3K27me3 levels ( Supplementary Fig. 3 ), suggesting that Jmjd3 plays a specific role in Shh target gene activation. RNAi inhibition of Jmjd3 expression in MEFs phenocopied the Jmjd3 −/− defects in Shh-induced Gli1 expression and local H3K27me3 reduction ( Supplementary Fig. 4 ). Notably, lack of another H3K27me3 demethylase, UTX [27] , did not produce significant effects on Shh-induced target gene expression in MEFs ( Supplementary Fig. 5 ). These results indicate that H3K27me3 and PRC2 are required for the repression of Shh target gene basal expression and that erasure of the mark by Jmjd3 in response to Shh is required for gene activation. Shh induces a local epigenetic switch from PRC2 to Jmjd3 We next monitored the dynamic binding of PRC2 and Jmjd3 in response to Shh signalling. In the Gli1 gene, a cluster of Gli-binding sites [30] , [31] overlaps the H3K27me3-enriched region ( Supplementary Fig. 6A ). Using ChIP, we demonstrated that endogenous SUZ12 and, by inference, PRC2, binds to Gli1 ; binding decreased on Shh treatment ( Fig. 2a ). Conversely, ChIP with a Jmjd3 antibody indicated increased binding of Jmjd3 to the Gli1 regulatory region on Shh induction ( Fig. 2b ). A ChIP experiment performed in NIH3T3 cells expressing FLAG-tagged Jmjd3 or HA-tagged EZH2 confirmed the binding dynamics: Shh treatment reduced EZH2 binding and increased Jmjd3 binding to Gli1 ( Supplementary Fig. S6 ). In MEFs, levels of EZH2, SUZ12 and Jmjd3 were similar with or without Shh treatment ( Fig. 2c,d ). Thus, the Shh-induced switch from PRC2 to Jmjd3 in these regulatory regions was not due to changes in the global levels of these factors but was likely caused by an active recruitment of Jmjd3 to replace PRC2 on Shh stimulation. Indeed, in the absence of Jmjd3, a significant amount of SUZ12 remained bound to Gli1 in Shh-treated cells ( Fig. 2a ), suggesting that Jmjd3 is required for removal of PRC2 from Shh target genes. 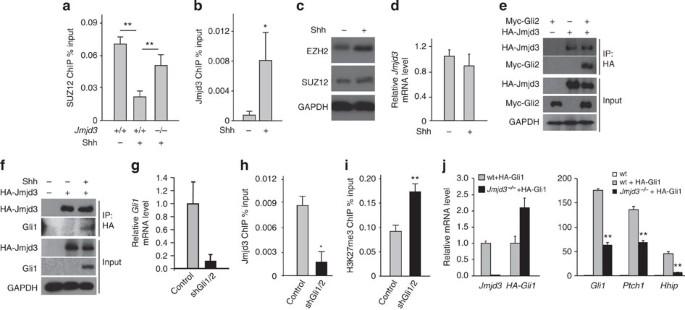Figure 2: Shh induces a Gli-dependent local epigenetic switch from PRC2 to Jmjd3. (a) ChIP-qPCR indicates the dynamic binding of endogenous SUZ12 to theGli1regulatory region in wild-type andJmjd3−/−MEF cells on Shh induction. (means±s.d.,n=3). (b) Increased Jmjd3 binding toGli1gene on Shh treatment was shown by ChIP-qPCR (means±s.d.,n=3). (c) Shh treatment did not reduce levels of PRC2 subunits as shown by EZH2 and SUZ12 western blot. (d)Jmjd3expression level was not significantly changed in MEFs by Shh treatment as analysed by RT–qPCR (means±s.d.,n=3). (e) Jmjd3 co-immunoprecipitates with Gli2. Lysates of NIH3T3 cells transiently transfected with plasmids expressing HA-Jmjd3 and Myc-Gli2 were immunoprecipitated with anti-HA antibodies and blotted with antibodies against HA and Myc. (f) Jmjd3 co-immunoprecipitates with endogenous Gli1. Cell lysates of Shh-treated NIH3T3 cells expressing HA-Jmjd3 were immunoprecipitated with anti-HA antibodies and blotted with antibodies against HA and Gli1. (g) RNAi-induced inhibition ofGli1andGli2in Shh-treated MEFs led to (h) decreased Jmjd3 binding and (i) increased H3K27me3 levels in theGli1regulatory region (means±s.d.,n=3). (j) Deletion ofJmjd3in MEFs led to impaired endogenous Shh target gene (Gli1, Ptch1, Hhip) expression induced by lentiviral expressed HA-Gli1 as shown by RT–qPCR. Expressions of endogenousGli1and exogenousHA-Gli1were measured using primers specific for the 5′-UTR and the HA tag region, respectively. Significance was determined usingt-test or ANOVA withpost hoc t-test (means±s.d.,n=3). ** indicatesP<0.01 and * indicatesP<0.05. Figure 2: Shh induces a Gli-dependent local epigenetic switch from PRC2 to Jmjd3. ( a ) ChIP-qPCR indicates the dynamic binding of endogenous SUZ12 to the Gli1 regulatory region in wild-type and Jmjd3 −/− MEF cells on Shh induction. (means±s.d., n =3). ( b ) Increased Jmjd3 binding to Gli1 gene on Shh treatment was shown by ChIP-qPCR (means±s.d., n =3). ( c ) Shh treatment did not reduce levels of PRC2 subunits as shown by EZH2 and SUZ12 western blot. ( d ) Jmjd3 expression level was not significantly changed in MEFs by Shh treatment as analysed by RT–qPCR (means±s.d., n =3). ( e ) Jmjd3 co-immunoprecipitates with Gli2. Lysates of NIH3T3 cells transiently transfected with plasmids expressing HA-Jmjd3 and Myc-Gli2 were immunoprecipitated with anti-HA antibodies and blotted with antibodies against HA and Myc. ( f ) Jmjd3 co-immunoprecipitates with endogenous Gli1. Cell lysates of Shh-treated NIH3T3 cells expressing HA-Jmjd3 were immunoprecipitated with anti-HA antibodies and blotted with antibodies against HA and Gli1. ( g ) RNAi-induced inhibition of Gli1 and Gli2 in Shh-treated MEFs led to ( h ) decreased Jmjd3 binding and ( i ) increased H3K27me3 levels in the Gli1 regulatory region (means±s.d., n =3). ( j ) Deletion of Jmjd3 in MEFs led to impaired endogenous Shh target gene ( Gli1, Ptch1, Hhip ) expression induced by lentiviral expressed HA-Gli1 as shown by RT–qPCR. Expressions of endogenous Gli1 and exogenous HA-Gli1 were measured using primers specific for the 5′-UTR and the HA tag region, respectively. Significance was determined using t -test or ANOVA with post hoc t -test (means±s.d., n =3). ** indicates P <0.01 and * indicates P <0.05. Full size image Shh-induced Gli1/2 activation and binding to target genes may mediate Jmjd3 recruitment. Gli2 and Shh-induced Gli1 both can co-immunoprecipitate with Jmjd3 ( Fig. 2e,f , Supplementary Fig. 7 ). The exogenous tagged Jmjd3 proteins are expressed in NIH3T3 cells at relatively low levels, as it is difficult to detect the full-length Jmjd3 proteins with standard western blot. Importantly, RNAi inhibition of Gli1/2 in Shh-treated MEF cultures ( Fig. 2g ) reduced Jmjd3 binding to the Gli1 regulatory region ( Fig. 2h ) and increased local H3K27me3 levels ( Fig. 2i ), suggesting that Gli1/2 are required for Jmjd3 binding to Shh target genes. In contrast, Gli1/2 binding to Shh target genes was not affected by Jmjd3 deletion ( Supplementary Fig. 8 ). Thus, Gli1/2 activators are required for the recruitment of Jmjd3 and possibly other coactivators to displace PRC2 and activate target gene expression. To further confirm that Jmjd3 directly regulates Gli-mediated transcription, we expressed HA-Gli1 in MEFs and observed that the activation of endogenous Gli target genes by HA-Gli1 was significantly impaired in Jmjd3 −/− MEFs compared with that in wild-type cells ( Fig. 2j ). Shh-induced switch is essential for target gene expression To determine whether the Shh-induced, Gli-mediated PRC2 to Jmjd3 switch is required for proper target gene expression, we manipulated local PRC2 and Jmjd3 levels to perturb the epigenetic switch, either by increasing local PRC2 levels after Shh treatment or introducing Jmjd3 onto the Gli1 gene before Shh stimulation. All three Gli proteins contain five conserved zinc-fingers that are sufficient to bind specifically to the Gli consensus sequence [38] . We fused the Gli3 DNA binding domain (GliDBD) to HA-tagged EZH2 and expressed this fusion in either NIH3T3 cells or MEF cells ( Fig. 3a , Supplementary Fig. 9A ). GliDBD-EZH2 interacted with endogenous SUZ12 as the two proteins were co-immunoprecipitated ( Fig. 3b ), suggesting that these proteins form a functional PRC2 complex. In the presence of Shh, GliDBD-EZH2 can bind Gli1 and increase local H3K27me3 levels as shown by ChIP ( Fig. 3c,d , Supplementary Fig. 9B,C ). Both GliDBD-EZH2 and exogenous EZH2 reduced Shh-activated Gli1 expression ( Fig. 3e , Supplementary Fig. 9D ). GliDBD-EZH2 repressed Gli1 more effectively and specifically than EZH2; EZH2 also repressed another Shh-independent target gene HoxA10 ( Fig. 3e , Supplementary Fig. 9D ). Thus, increasing the local PRC2 concentration in Shh-stimulated conditions effectively repressed Gli1 expression, indicating that PRC2 must be removed to activate gene expression. Using similar approaches, we found that GliDBD-Jmjd3 expressed in NIH3T3 cells ( Fig. 3f ) bound to the Shh target gene regulatory regions under basal conditions ( Fig. 3g ) and decreased local H3K27me3 ( Fig. 3h ). GliDBD-Jmjd3 activated Shh target genes even in the absence of Shh stimulation ( Fig. 3i ). Thus, recruitment of Jmjd3 is sufficient to increase Gli target gene expression before Shh stimulation. These data indicate that the presence of PRC2 represses the expression of Shh target genes, whereas the removal of PRC2 and the recruitment of Jmjd3 on Shh stimulation activate gene expression. Thus, the Shh-induced epigenetic switch from PRC2 to Jmjd3 is essential for target gene activation. 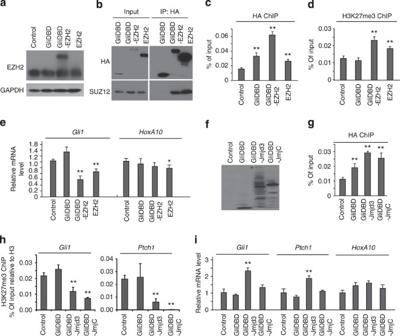Figure 3: The Shh-induced local PRC2 to Jmjd3 switch is essential for proper target gene expression. (a) Total EZH2 levels in NIH3T3 cells expressing the indicated exogenous proteins as shown by western blot with anti-EZH2 antibodies. (b) Exogenous EZH2 and GliDBD-EZH2, but not GliDBD, expressed in NIH3T3 cells interact with endogenous SUZ12 as indicated by IP with an HA antibody and western blot with SUZ12 antibody. All exogenous proteins contain an HA tag. (c) GliDBD-EZH2 proteins are recruited toGli1regulatory region as indicated by ChIP-qPCR with anti-HA antibodies (means±s.d.,n=3). (d) Local H3K27me3 levels atGli1regulatory region as measured by ChIP-qPCR in Shh-treated NIH3T3 cells expressing exogenous proteins (means±s.d.,n=3). (e) RT–qPCR analyses ofGli1andHoxA10in Shh-treated NIH3T3 cells expressing the indicated exogenous proteins (means±s.d.,n=3). (f) Expression of fused Jmjd3 proteins in transfected NIH3T3 cells detected by western blot using anti-HA antibodies. The full-length GliDBD-Jmjd3 protein band is marked with a star. (g) Binding of HA-tagged GliDBD fusion Jmjd3 proteins and (h) local H3K27me3 levels atGli1andPtch1loci as shown by ChIP-qPCR. Histone H3 ChIP was used for normalization (means±s.d.,n=3). (i) RT–qPCR analyses ofGli1,Ptch1andHoxA10in NIH3T3 cells expressing the indicated exogenous Jmjd3 proteins in basal conditions (means±s.d.,n=3). Significance was determined usingt-test or ANOVA withpost hoc t-test; ** indicatesP<0.01 and * indicatesP<0.05. The comparisons are all against the control samples. Figure 3: The Shh-induced local PRC2 to Jmjd3 switch is essential for proper target gene expression. ( a ) Total EZH2 levels in NIH3T3 cells expressing the indicated exogenous proteins as shown by western blot with anti-EZH2 antibodies. ( b ) Exogenous EZH2 and GliDBD-EZH2, but not GliDBD, expressed in NIH3T3 cells interact with endogenous SUZ12 as indicated by IP with an HA antibody and western blot with SUZ12 antibody. All exogenous proteins contain an HA tag. ( c ) GliDBD-EZH2 proteins are recruited to Gli1 regulatory region as indicated by ChIP-qPCR with anti-HA antibodies (means±s.d., n =3). ( d ) Local H3K27me3 levels at Gli1 regulatory region as measured by ChIP-qPCR in Shh-treated NIH3T3 cells expressing exogenous proteins (means±s.d., n =3). ( e ) RT–qPCR analyses of Gli1 and HoxA10 in Shh-treated NIH3T3 cells expressing the indicated exogenous proteins (means±s.d., n =3). ( f ) Expression of fused Jmjd3 proteins in transfected NIH3T3 cells detected by western blot using anti-HA antibodies. The full-length GliDBD-Jmjd3 protein band is marked with a star. ( g ) Binding of HA-tagged GliDBD fusion Jmjd3 proteins and ( h ) local H3K27me3 levels at Gli1 and Ptch1 loci as shown by ChIP-qPCR. Histone H3 ChIP was used for normalization (means±s.d., n =3). ( i ) RT–qPCR analyses of Gli1 , Ptch1 and HoxA10 in NIH3T3 cells expressing the indicated exogenous Jmjd3 proteins in basal conditions (means±s.d., n =3). Significance was determined using t -test or ANOVA with post hoc t -test; ** indicates P <0.01 and * indicates P <0.05. The comparisons are all against the control samples. Full size image Coordinated target gene activation by Jmjd3 and Set1/MLL Our results indicate that Jmjd3 is required for the removal of H3K27me3 and activation of Shh target genes. It is not clear whether its demethylase activity is essential and/or sufficient for this function. The C-terminal fragment of Jmjd3, encompassing the JmjC domain, is sufficient to catalyse H3K27me3 demethylation and rescues several Jmjd3-deficient phenotypes [21] , [25] . The expression of the C-terminal fragment (aa 1,141–1,641) fused with GliDBD (GliDBD-JmjC) was sufficient to reduce local H3K27me3 levels at Gli1 locus ( Fig. 3g,h ), but it did not activate Shh target gene basal expression ( Fig. 3i ). Thus, the Jmjd3 enzymatic activity alone is not sufficient to activate Shh target genes. We performed rescue experiments in NIH3T3 cells co-expressing an shRNA targeting Jmjd3 and exogenous RNAi-resistant genes encoding Jmjd3, the JmjC domain, or the Jmjd3-H1388A enzymatically inactive proteins [21] . The cultures were co-transfected with plasmids expressing GFP-Gli1 to activate the endogenous Shh target genes ( Fig. 4a,b ). Although each of these Jmjd3 proteins bound to the Gli1 regulatory region ( Fig. 4c ), only wild-type full-length Jmjd3 rescued the defective Gli1-induced gene expression in Jmjd3 -knockdown cells ( Fig. 4a ), indicating that the demethylase activity is necessary but not sufficient for activation of Gli target genes. The non-enzymatic activity of Jmjd3 may serve to recruit other epigenetic regulators. 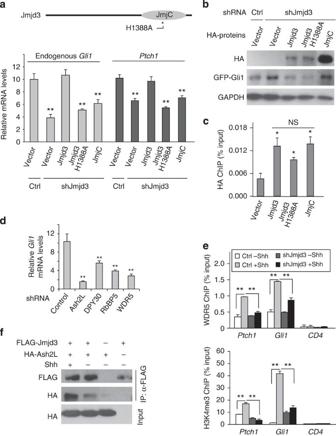Figure 4: Coordinated functions of Jmjd3 and Set1/MLL regulate Shh-activated gene transcription. (a) Both the enzymatic and non-enzymatic activities of Jmjd3 are required for its function in Shh-induced gene activation. NIH3T3 cells infected withJmjd3shRNA or vector control were transfected with plasmids co-expressing GFP-Gli1 and indicated Jmjd3 proteins or vector controls. Levels of endogenousGli1andPtch1were determined by RT–qPCR (means±s.d.,n=3). (b) Expression of HA-tagged Jmjd3 proteins and exogenous GFP-Gli1 levels in transfected cells as detected by western blot. (c) Binding of Jmjd3 and mutants toGli1regulatory region was determined by HA ChIP-qPCR. ‘NS’ indicates not significant (means±s.d.,n=3). (d) Set1/MLL complexes are important for Shh-induced target gene activation. RNAi-mediated inhibition of expression of individual Set1/MLL subunitsAsh2L,DPY30,RbBP5andWDR5significantly impairedGli1expression in the presence of Shh as measured by RT–qPCR (means±s.d.,n=3). (e) Shh-induced binding of WDR5 to Shh target genes requires the presence of Jmjd3. Shown are ChIP-qPCR analyses with antibodies against endogenous WDR5 and H3K4me3 in NIH3T3 cells expressing shRNA targetingJmjd3or scrambled shRNA in the basal or Shh-treated conditions.CD4was the negative control (means±s.d.,n=3). (f) Shh enhances the interactions between Jmjd3 and Set1/MLL subunits. NIH3T3 cells co-transfected with plasmids expressing FLAG-Jmjd3 and HA-Ash2L were treated with or without Shh. An anti-FLAG antibody was used for immunoprecipitation, and antibodies against FLAG or HA were used for western blot. Significance was determined usingt-test or ANOVA withpost hoc t-test; ** indicatesP<0.01 and * indicatesP<0.05. The comparisons are all against the control samples. Figure 4: Coordinated functions of Jmjd3 and Set1/MLL regulate Shh-activated gene transcription. ( a ) Both the enzymatic and non-enzymatic activities of Jmjd3 are required for its function in Shh-induced gene activation. NIH3T3 cells infected with Jmjd3 shRNA or vector control were transfected with plasmids co-expressing GFP-Gli1 and indicated Jmjd3 proteins or vector controls. Levels of endogenous Gli1 and Ptch1 were determined by RT–qPCR (means±s.d., n =3). ( b ) Expression of HA-tagged Jmjd3 proteins and exogenous GFP-Gli1 levels in transfected cells as detected by western blot. ( c ) Binding of Jmjd3 and mutants to Gli1 regulatory region was determined by HA ChIP-qPCR. ‘NS’ indicates not significant (means±s.d., n =3). ( d ) Set1/MLL complexes are important for Shh-induced target gene activation. RNAi-mediated inhibition of expression of individual Set1/MLL subunits Ash2L , DPY30 , RbBP5 and WDR5 significantly impaired Gli1 expression in the presence of Shh as measured by RT–qPCR (means±s.d., n =3). ( e ) Shh-induced binding of WDR5 to Shh target genes requires the presence of Jmjd3. Shown are ChIP-qPCR analyses with antibodies against endogenous WDR5 and H3K4me3 in NIH3T3 cells expressing shRNA targeting Jmjd3 or scrambled shRNA in the basal or Shh-treated conditions. CD4 was the negative control (means±s.d., n =3). ( f ) Shh enhances the interactions between Jmjd3 and Set1/MLL subunits. NIH3T3 cells co-transfected with plasmids expressing FLAG-Jmjd3 and HA-Ash2L were treated with or without Shh. An anti-FLAG antibody was used for immunoprecipitation, and antibodies against FLAG or HA were used for western blot. Significance was determined using t -test or ANOVA with post hoc t -test; ** indicates P <0.01 and * indicates P <0.05. The comparisons are all against the control samples. Full size image Activation of bivalent genes is accompanied by coordinated changes in levels of both H3K27me3 and H3K4me3. Thus, it is likely that Jmjd3 and the Set1/MLL family of H3K4me3 methyltransferase complexes function cooperatively to regulate Shh-induced gene activation. Ash2L, RbBP5, DPY30 and WDR5 are essential subunits for all Set1/MLL family complexes [39] . RNAi inhibition of expression of individual subunits significantly impaired Gli1 expression in Shh-treated NIH3T3 cells ( Fig. 4d ). To determine whether Shh signalling regulates Set1/MLL complex binding to Shh target genes, we performed ChIP with WDR5 antibodies. Consistent with the Shh-induced increase of local H3K4me3, the binding of endogenous WDR5 to Gli1 and Ptch1 regulatory regions was significantly increased on Shh treatment ( Fig. 4e ). Importantly, in cells deficient in Jmjd3, Shh-induced WDR5 binding to target genes and local H3K4me3 increases were significantly impaired ( Fig. 4e ). Consistent with this result, local levels of H3K4me3 in the Gli1 gene in the presence of Shh were significantly lower in Jmjd3 −/− MEFs than in wild-type cells ( Supplementary Fig. 10 ). Thus, Jmjd3 is required for Set1/MLL complexes recruitment to target genes in response to Shh stimulation. It is not clear whether the interaction between Jmjd3 and Set1/MLL complexes [21] plays a role in resolving bivalent domains; however, our co-immunoprecipitation analyses showed that interactions between Jmjd3 and Set1/MLL subunits, WDR5 and ASH2L, were significantly enhanced by Shh stimulation ( Fig. 4f , Supplementary Fig. 11 ). The Shh-induced JmjD3–MLL interaction is potentially phosphorylation-dependent, as treating the lysate with λ -phosphatase reduced the interaction to the basal level ( Supplementary Fig. 11 ). This result suggests that Shh signalling directly modulates epigenetic complexes required for target gene activation. Thus, in addition to the PRC2 to Jmjd3 switch, Shh signalling also induces the formation of an epigenetic coactivator complex containing at least Jmjd3 and Set1/MLL, which regulates target gene activation coordinately by modulating the bivalent domains. Jmjd3 −/− mice display Shh-dependent developmental defects As Jmjd3 is a key factor in Shh-induced epigenetic switch and gene activation, we examined its function in Shh-activation-dependent developmental processes. As shown by analysis of Gli2 −/− mice, Gli2-mediated Shh activation is required for multiple developmental processes such as hair follicle development, ventral neural tube patterning and cerebellum progenitor proliferation [8] , [40] , [41] , [42] . Like Gli2 −/− mice, Jmjd3 −/− mice die at birth due to respiratory failure [24] , [25] , [43] . Interestingly, Jmjd3 −/− mice display multiple defects similar to Gli2 −/− mice in Shh/Gli2-dependent developmental processes. As a morphogen, Shh is important for neural tube patterning and neural progenitor specification. During neural tube development, Shh mainly functions to antagonize GliR activity, whereas GliA is only required for the formation of the floor plate and specification of the most ventral neural progenitors [6] , [7] . Gli2 −/− neural tubes display reduced expression of markers for floor plate and V3 interneuron progenitors [40] , [41] . Jmjd3 is expressed in the ventral neural tube but not in the floor plate [44] . In E10.5 Jmjd3 −/− neural tubes, V3 interneuron progenitor marker Nkx2.2 levels were significantly reduced ( Supplementary Fig. 12A,A′,C,C′,F ) and Olig2-expressing motor neuron progenitor regions were expanded ( Supplementary Fig. 12B,B′,C,C′,F ). These defects are similar to those observed in Gli2 −/− embryos [40] . We also observed a reduction of FoxA2 expression in Jmjd3 −/− neural tubes but not in the floor plate ( Supplementary Fig. 12D,D′ ), possibly due to the absence of Jmjd3 in the floor plate or the usage of alternative activation mechanisms. The enriched expression of Ptch1 in the most ventral neural tubes was also reduced in Jmjd3 −/− embryos ( Supplementary Fig. 12E,E′ ). Thus, these results are consistent with a function of Jmjd3 in GliA-dependent target gene expression and ventral neural tube development. Shh-dependent Gli2 activation is essential for embryonic hair follicle development. Gli2 −/− embryos exhibit an arrest in hair follicle development with reduced cell proliferation [42] . When hair follicles in the sections of E18.5 Jmjd3 −/− skin were analysed, we observed similarly delayed development of hair follicles. Although both control (wild type and Jmjd3 +/− ) and Jmjd3 −/− skins contain hair follicles from all stages [45] (stage 1 to 5, Supplementary Fig. 13A–D ), Jmjd3 −/− hair follicles were arrested at earlier developmental stages with a peak at stage 2 ( Supplementary Fig. 13E ). Control hair follicles grew deeper and had more mature morphologies with a peak at stage 3 ( Supplementary Fig. 13E ). This defect in Shh/GliA-dependent hair follicle development further corroborates the importance of Jmjd3 in Shh signalling activation. Jmjd3 is required for Shh-dependent CGNP proliferation During cerebellum development from late embryonic to the early postnatal stage (E18.5–P14), CGNPs in the external granule layer (EGL) undergo significant expansion and differentiation into granule neurons, the most abundant neuron type in the nervous system. Multiple signalling pathways and transcription factors coordinate to regulate this process, and Shh-mediated Gli activation is necessary for CGNP proliferation [9] , [10] , [11] . Interestingly, during the period from E16.5 to P5, there is a global decrease of H3K27me3 and increase of H3K4me3 and H3K27Ac in the cerebellum ( Fig. 5a ). The decrease of global H3K27me3 levels was apparent in EGL CGNPs ( Fig. 5b ) and correlated with the expression of a large amount of genes required for rapid expansion and differentiation of CGNPs at P5. Specifically, at Shh target genes, the activation of Gli1 expression at P5 was accompanied by a decrease of H3K27me3 and an increase of H3K4me3 ( Fig. 5c ), which is similar to the signalling-induced resolution of the bivalent domain in MEFs. These data suggest that the Shh-induced epigenetic switch also occurs in the developing cerebellum to modulate the bivalent domain and activate target genes, which contributes to the global change of H3K27me3 levels. 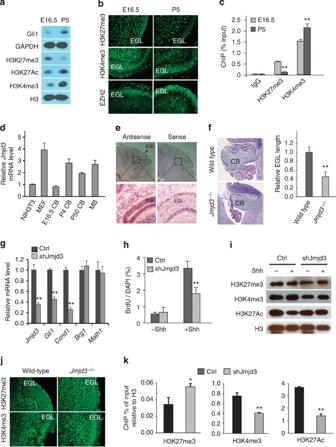Figure 5: Jmjd3 is required for Shh-dependent CGNP proliferation. (a) Global changes of modified histone levels during cerebellum development evaluated by western blot. (b) Immunostaining of sections of E16.5 and P5 cerebella with antibodies against modified histones and EZH2. The EGL is the dense cell layer outlining the cerebellum. (c) Local changes of H3H27me3 and H3K4me3 atGli1regulatory region in E16.5 and P5 cerebella (means±s.d.,n=3). (d) RT–qPCR analysis ofJmjd3in NIH3T3 and MEF cells and in cerebellum (CB) and medulloblastoma (MB) samples (means±s.d.,n=3). (e)In situhybridization of P5 CB withJmjd3antisense or sense probes. Note the enriched Jmjd3 expression in EGL. (f) H&E staining of cerebella from E18.5 wild-type andJmjd3−/−mice. The average length of EGL per cerebellum section is shown on the right (means±s.d.,n=4). (g) Inhibition ofJmjd3expression in cultured CGNPs results in defective Shh-induced gene expression as shown by RT–qPCR. (h)Jmjd3knockdown in cultured CGNPs decreases proliferation (as shown by BrdU incorporation) (means±s.d.,n=3). (i) Western blots indicating global histone modification levels in CGNP cultures in the absence and presence of Shh treatment with or withoutJmjd3shRNA treatment. (j) Immunostaining of sections of E18.5 wild-type andJmjd3−/−cerebella with antibodies against modified histones. (k) Decrease inJmjd3levels in Shh-treated CGNP cultures by lentiviral-expressed shRNA resulted in significant changes of histone modifications at theGli1regulatory region as shown by ChIP-qPCR. Histone H3 ChIP was used for normalization (means±s.d.,n=3). Significance was determined by Student’st-test; ** indicatesP<0.01 and * indicatesP<0.05. Figure 5: Jmjd3 is required for Shh-dependent CGNP proliferation. ( a ) Global changes of modified histone levels during cerebellum development evaluated by western blot. ( b ) Immunostaining of sections of E16.5 and P5 cerebella with antibodies against modified histones and EZH2. The EGL is the dense cell layer outlining the cerebellum. ( c ) Local changes of H3H27me3 and H3K4me3 at Gli1 regulatory region in E16.5 and P5 cerebella (means±s.d., n =3). ( d ) RT–qPCR analysis of Jmjd3 in NIH3T3 and MEF cells and in cerebellum (CB) and medulloblastoma (MB) samples (means±s.d., n =3). ( e ) In situ hybridization of P5 CB with Jmjd3 antisense or sense probes. Note the enriched Jmjd3 expression in EGL. ( f ) H&E staining of cerebella from E18.5 wild-type and Jmjd3 −/− mice. The average length of EGL per cerebellum section is shown on the right (means±s.d., n =4). ( g ) Inhibition of Jmjd3 expression in cultured CGNPs results in defective Shh-induced gene expression as shown by RT–qPCR. ( h ) Jmjd3 knockdown in cultured CGNPs decreases proliferation (as shown by BrdU incorporation) (means±s.d., n =3). ( i ) Western blots indicating global histone modification levels in CGNP cultures in the absence and presence of Shh treatment with or without Jmjd3 shRNA treatment. ( j ) Immunostaining of sections of E18.5 wild-type and Jmjd3 −/− cerebella with antibodies against modified histones. ( k ) Decrease in Jmjd3 levels in Shh-treated CGNP cultures by lentiviral-expressed shRNA resulted in significant changes of histone modifications at the Gli1 regulatory region as shown by ChIP-qPCR. Histone H3 ChIP was used for normalization (means±s.d., n =3). Significance was determined by Student’s t -test; ** indicates P <0.01 and * indicates P <0.05. Full size image Despite the low global level of H3K27me3, EZH2 protein levels remained high in P5 CGNPs ( Fig. 5b ), suggesting that a high level of H3K27me3 demethylase activity is present. We observed that Jmjd3 expression was increased during cerebellar development from E16.5 to P4 ( Fig. 5d ). In P5 cerebellum, Jmjd3 was enriched in EGL ( Fig. 5e ). Interestingly, at E18.5, Jmjd3 −/− mice displayed decreased cerebellum size and lack of foliation ( Fig. 5f ), which are similar to the defects observed in the Gli2 −/− cerebellum [8] and are likely caused by impaired CGNP proliferation. To directly determine the function of Jmjd3 in CGNP proliferation, we inactivated Jmjd3 using RNAi in Shh-treated P4 CGNP cultures. Reduction of Jmjd3 levels in CGNPs significantly impaired the expression of Shh-induced genes such as Gli1 and mitogenic Ccnd1 but not other genes such as Brg1 and the CGNP marker Math1 ( Fig. 5g ). The proliferation of CGNPs in which Jmjd3 expression was inhibited was significantly impaired as shown by the lower BrdU incorporation rates compared with control cultures ( Fig. 5h ). Although neither Shh treatment nor Jmjd3 inhibition in CGNPs led to global changes of histone modifications, we observed altered H3K27me3 as well as H3K4me3 and H3K27Ac levels at Gli1 regulatory regions in Shh-treated Jmjd3 -deficient cultures compared with the controls ( Fig. 5i–k ). A Cre-induced Jmjd3 conditional deletion [46] in CGNP cultures displayed similar defects in Shh target gene expression and altered histone modifications ( Supplementary Fig. 14 ). Thus, Jmjd3 regulates Shh-activated gene expression and CGNP proliferation by modulating the chromatin environment. Inhibition of Jmjd3 impairs medulloblastoma cell growth Mutations leading to constitutively active Shh signalling cause Shh-subtype medulloblastoma, the progression of which also requires the active signalling pathway [4] , [47] . Thus, as a key epigenetic coactivator of Shh target genes, Jmjd3 might be targeted to inhibit medulloblastoma growth. We used a mouse model with a Cre-inducible SmoM2 gene (a point mutation in Smo ) to generate Shh-subtype medulloblastoma [48] ( Fig. 6a ). SmoM2-induced medulloblastoma cells contain much lower H3K27me3 levels than normal cerebellar tissues ( Fig. 6b,c ). As a significant amount of EZH2 was expressed in SmoM2-induced medulloblastoma ( Fig. 6b–d ), the low H3K27me3 levels suggest that H3K27me3 demethylase is active in these tumour cells. Notably, although Jmjd3 is mutated in some cancers and even in non-Shh-type medulloblastoma [47] , [49] , it has not been found mutated in Shh-type medulloblastoma in several genome-wide exome-sequencing projects [47] , [50] , [51] , [52] , [53] , indicating a potential requirement of Jmjd3 for these tumours. 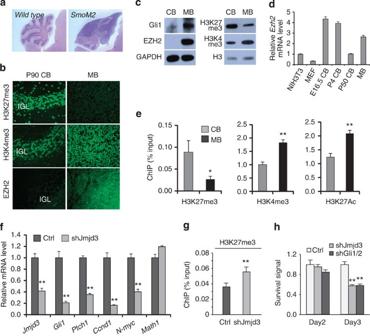Figure 6: Jmjd3 is required for Shh-subtype medulloblastoma cell growth. (a) H&E staining of sections of a P90 normal cerebellum and one with a SmoM2-induced MB. (b) Levels of histone modifications and EZH2 in normal cerebellum (CB) and SmoM2-induced medulloblastoma (MB) were analysed by immunostaining. IGL=internal granule layers. (c) Western blots indicating global levels of histone modifications and EZH2 in normal CB and SmoM2 MB. (d) RT–qPCR analysis ofEZH2in NIH3T3 and MEF cells and in CB and MB samples (means±s.d.,n=3). (e) ChIP-qPCR analysis of histone modification levels in theGli1regulatory region in MB and normal CB. Histone H3 ChIP was used for ChIP normalization. (means±s.d.,n=3). (f) Cultured SmoM2 medulloblastoma tumour cells were infected with lentiviruses expressing eitherJmjd3shRNA or scrambled control. Levels of Shh target genes and medulloblastoma progenitor markerMath1were measured with RT–qPCR (means±s.d.,n=3). (g) The H3K27me3 level in theGli1gene regulatory region was increased after inhibition ofJmjd3expression (means±s.d.,n=3). (h) Cultured SmoM2 tumour cells were infected with viruses expressing control or shRNA targetingJmjd3orGli1/2. The survival rates of cells relative to the control culture were measured using the ATP cell viability assay (means±s.d.,n=3). Significance was determined by Student’st-test or ANOVA withpost hoc t-test; ** indicatesP<0.01 and * indicatesP<0.05. Figure 6: Jmjd3 is required for Shh-subtype medulloblastoma cell growth. ( a ) H&E staining of sections of a P90 normal cerebellum and one with a SmoM2-induced MB. ( b ) Levels of histone modifications and EZH2 in normal cerebellum (CB) and SmoM2-induced medulloblastoma (MB) were analysed by immunostaining. IGL=internal granule layers. ( c ) Western blots indicating global levels of histone modifications and EZH2 in normal CB and SmoM2 MB. ( d ) RT–qPCR analysis of EZH2 in NIH3T3 and MEF cells and in CB and MB samples (means±s.d., n =3). ( e ) ChIP-qPCR analysis of histone modification levels in the Gli1 regulatory region in MB and normal CB. Histone H3 ChIP was used for ChIP normalization. (means±s.d., n =3). ( f ) Cultured SmoM2 medulloblastoma tumour cells were infected with lentiviruses expressing either Jmjd3 shRNA or scrambled control. Levels of Shh target genes and medulloblastoma progenitor marker Math1 were measured with RT–qPCR (means±s.d., n =3). ( g ) The H3K27me3 level in the Gli1 gene regulatory region was increased after inhibition of Jmjd3 expression (means±s.d., n =3). ( h ) Cultured SmoM2 tumour cells were infected with viruses expressing control or shRNA targeting Jmjd3 or Gli1/2 . The survival rates of cells relative to the control culture were measured using the ATP cell viability assay (means±s.d., n =3). Significance was determined by Student’s t -test or ANOVA with post hoc t -test; ** indicates P <0.01 and * indicates P <0.05. Full size image To determine the function of Jmjd3 in medulloblastoma, we first confirmed that in SmoM2 medulloblastoma the Gli1 regulatory regions contain lower H3K27me3 levels and higher H3K4me3 and H3K27Ac levels than normal cerebellum ( Fig. 6e ). Reducing Jmjd3 expression using virally expressed shRNA significantly impaired the expression of Shh target genes such as Gli1 , Ptch1 , Ccnd1 and N-myc in cultured SmoM2 tumour cells ( Fig. 6f ). This defect was not due to the differentiation of tumour cells because the tumour progenitor marker Math1 was not significantly reduced ( Fig. 6f ). Local H3K27me3 levels on the Gli1 gene were significantly increased on inhibition of Jmjd3 expression ( Fig. 6g ). The impaired Shh target gene expression in Jmjd3-deficient tumour cells led to a growth inhibition similar to that observed in Gli1/2-deficient tumour cultures as indicated by a cell survival assay ( Fig. 6h ). Therefore, as Jmjd3 is required for Shh-subtype medulloblastoma growth, Shh-induced epigenetic switching events may be targeted to inhibit medulloblastoma growth. In this report, we have identified a bivalent chromatin domain tightly associated with the poised states of Shh target genes. We have shown that Shh signalling induces a local epigenetic switch as well as the formation of a Jmjd3-centred epigenetic coactivator complex, which functions coordinately with GliA to resolve the bivalent domain and to activate transcription. We have also demonstrated the essential role of Jmjd3 in regulating Shh-dependent developmental processes and tumour proliferation. The epigenetic mechanisms elucidated here significantly advance our understanding of Shh signalling and provide insights into the mechanisms of Shh-related cancers and diseases. Activation of Shh signalling induces a local epigenetic switch from PRC2 to Jmjd3 at Shh target genes to facilitate the resolution of bivalent chromatin domains. The removal of H3K27me3 in response to Shh likely resulted from both the recruitment of Jmjd3 and the release of PRC2. We propose that, on Shh signalling stimulation, the activation and binding of Gli1/2 mediate the recruitment of Jmjd3 and subsequently the coactivator complex, which displaces PRC2 at the regulatory regions, resolves bivalent domains and activates target genes ( Supplementary Fig. 16 ). In the absence of Jmjd3, GliA binding was not affected, but PRC2 release was impaired and Set1/MLL was not recruited. Although Jmjd3 also functions in other pathways, in tissues that are predominantly dependent on GliA function, such as embryonic hair follicle, ventral neural tube, cerebellum, and Shh-type medulloblastoma, inhibition of Jmjd3 expression and Gli2 deletion led to similar phenotypes. Thus, Jmjd3 plays an essential role in Shh-induced gene activation by coordinating the changes of chromatin environments. Shh signalling also significantly enhances the interactions between Jmjd3 and Set1/MLL complexes. Although the biochemical bases for this Shh-induced interaction remain unclear, the possibility that Shh signalling directly modifies epigenetic cofactors and regulate their activities is intriguing. Although the experiments were performed in populations of cells and we could not exclude the possibility that a fraction of the histone marks may exist in separate cells, our data strongly support the coexistence of H3K27me3 and H3K4me3 at the same loci and cooperative regulation of both marks by Shh signalling. The Shh-induced interaction between Jmjd3 and MLL suggests that they function together to regulate both histone marks. Importantly, loss of Jmjd3 not only affected the H3K27me3 levels at Gli target genes, but also impaired Shh-induced recruitment of Set1/MLL complexes and increase of H3K4me3 levels ( Fig. 4f ). In CGNPs, loss of Jmjd3 also affected the levels of both histone marks at Shh target genes ( Fig. 5k ). These results could unlikely be explained if the two histone marks are in separate cells and regulated independently. We propose that Shh-induced transcription factor exchange from GliR to GliA triggers the switch of the associated epigenetic complexes. Previous work and this report demonstrate that a complex epigenetic environment controls Shh target gene expression. It has been shown that Shh signalling also functions as switches for several epigenetic regulators that may coordinate with PRC2/Jmjd3 to regulate transcription outcomes. We have previously reported that Shh activation enables Brg1-containing BAF chromatin remodelling complexes to switch from a repressor to an activator state, a switch likely mediated by interacting with different Gli transcription factors and other epigenetic regulators [12] . Brg1 may either antagonize or facilitate PRC2 function in a context-dependent manner in embryonic stem cell gene expression [54] . Brg1 has also been shown to interact with Jmjd3 to induce specific target gene expression [55] . Thus, the Brg1 complex may coordinate with these histone modifiers to regulate Shh signalling. Indeed, deletion of Brg1 resulted in altered histone modifications (ref. 12 and our unpublished data). In addition, histone deacetylases (HDACs) and histone acetyl transferases (HATs) have been directly or indirectly linked to Shh signalling transcription regulation [12] , [56] , [57] , [58] . Interestingly, Shh signalling activities also alter HDAC function. In basal conditions, HDACs are likely involved in repressing the expression of Shh target genes by deacetylating histones [12] . However, on signal activation, HDAC1/2 function as activators of Shh target genes possibly by deacetylating and activating Gli1/2 (refs 12 , 56 ). HDACs have been shown to tightly interact with Brg1 as well as PRC2 complexes [12] , [59] . Deletion of the gene encoding PRC2 subunit EZH2 led to global increase of H3K27Ac [35] , [60] ( Supplementary Fig. 15 ). On Shh stimulation, the resolution of the bivalent domain is also accompanied with an increase of H3K27Ac at the regulatory regions ( Supplementary Fig. 2 ,). It is not clear whether the increased H3K27Ac is a byproduct of H3K27me3 loss or due to active recruitment of the H3K27 acetyltransferase p300/CBP [60] , [61] . In addition, Jmjd3 has been shown to interact with proteins involved in transcription elongation [62] , which may also function to regulate Shh signalling. During development, Shh can function as a mitogen or a morphogen. For the mitogenic function, Shh-induced GliA-mediated transcription activation is required. In this study, we demonstrated that during cerebellum development, when active Shh signalling plays an essential role in CGNP proliferation, Shh activation is accompanied by a decrease of H3K27me3 and an increase of H3K4me3 levels. Shh-subtype medulloblastomas are characterized by low levels of H3K27me3. We have shown that a key epigenetic factor Jmjd3 is required for the histone modification changes and Shh target gene activation in CGNPs and medulloblastoma cells. Deletion of Jmjd3 affects cerebellum growth and CGNP proliferation. Inhibiting enzymatic and/or non-enzymatic activities of Jmjd3 may effectively inhibit medulloblastoma growth. In addition to the mitogenic function, Shh also functions as a morphogen to induce dosage-dependent expression of target genes [2] . The diverse outputs of Shh signalling are thought to be determined by the combination of activities of GliA and GliR [6] , [7] , [63] . Thus, the mechanisms that underlie basal versus signalling-induced conditions identified here might also function in more complicated Shh-responsive systems. The morphogenic activities of Shh signalling are largely mediated by antagonizing GliR function [64] , [65] . We identified PRC2 as a corepressor of Shh target genes. However, we believe that PRC2 is only part of a complex corepressor network associated with GliR. GliA activities are required in the areas receiving highest Shh signalling. We also showed modest but significant defects in Jmjd3 −/− neural tubes in the most ventral area. Recent studies have revealed that the dosage-dependent transcription response to Shh results from different affinities for Gli-binding sites, other tissue-specific transcription factors, and functional interactions between different target genes [6] , [7] , [63] . It is likely that chromatin environment and epigenetic regulators also play important roles in determining the transcription outcomes of target genes in response to Shh. Additional genetic tools as well as more sensitive ChIP techniques will be needed to directly analyse the epigenetic regulation of the complex Shh-responsive systems. In summary, our study revealed a novel epigenetic mechanism that regulates Shh-induced gene activation. We identified Jmjd3 as a key regulator of Shh-activated gene expression and Shh-dependent developmental processes and tumour growth. In the future, the characterization of the components and analysis of the dynamics of epigenetic complexes downstream of Shh signalling will reveal the mechanisms underlying the diverse transcription activities of the signalling during development and in diseases. Mice Jmjd3 −/− MEFs were produced from E15.5 Jmjd3 −/− embryos [25] . This allele deletes exons 14–21, which encode a region that includes the JmjC demethylase domain. RT–PCR primers Jmjd3_koF1 and Jmjd3_koR1 ( Supplementary Information ) were used to detect the deletion of the Jmjd3 mRNA. E10.5 and E18.5 Jmjd3 −/− embryos were produced from mice containing a Jmjd3 / Kdm6b tm1(KOMP)Wtsi allele (Shpargel and Magnuson, unpublished data). This allele with exons 11–20 replaced by a Neo cassette was targeted by Knockout Mouse Project (KOMP) in JM8 embryonic stem cells of C57BL/6N origin. Embryonic stem cells were injected into C57BL/6J- Tyr c-2J /J blastocysts. Following germline transmission, mice were maintained on the C57BL/6J background. Homozygotes were generated by heterozygous intercrosses. Both Jmjd3 alleles delete a large portion of the protein, and these mice die at birth due to respiratory defects, which is similar to the phenotype of another Jmjd3 knockout allele [24] . Both alleles also result in similar skin and cerebellum defects at E18.5 and are likely null alleles. Jmjd3 conditional knockout allele was generated as previously described with exons 15 to 21 flanked by two LoxP sites [46] . SmoM2 mice [48] and CAG-CreER [66] mice were purchased from Jackson Laboratory. The SmoM2 CAG-CreER mice have a high rate of spontaneous medulloblastoma development before 2 months of age (~40%). These mice were maintained on a mixed genetic background at UT Southwestern Medical Center Animal Facility. Primary MEF, CGNP and medulloblastoma cell cultures Primary MEFs were cultured from E13.5 to E15.5 embryos as described previously [12] . In brief, embryo trunks were dissected, trypsinized, dissociated to single cells and cultured in DMEM media with 10% fetal bovine serum. Primary CGNP cultures were derived from dissociated P4 mouse cerebella and cultured in DMEM/F12 media containing 25 mM KCl, N 2 and 10% FBS. For Shh stimulation, Shh-conditioned medium produced from Shh-CM 293T cells [67] was added at a 1:20 dilution to MEF and CGNP cultures. MEF cells were treated with Shh in low-serum media 24 h before harvesting. CGNP cells were treated with Shh in high-serum media for 2–3 days. BrdU was added 2 h before analyses. Tumour cells were derived from dissociated SmoM2 medulloblastoma and cultured in the media containing DMEM/F12, B27, N2, EGF and FGF2. Plasmid construction, virus preparation and transfection/infection The shRNA sequences targeting Jmjd3 (5′- AGCACTCGATGCCTCATTCATA )-3′ (ref. 21 ), Ash2L (5′- CGAGTCTTGTTAGCCCTACAT -3′), DPY30 (5′- GCGTTGAGAGAATAGTCGAAA -3′), RbBP5 (5′- GCTCTATTGTATTTACCCATT -3′), WDR5 (5′- GCCGTTCATTTCAACCGTGAT -3′), Gli1 (5′- GCTCAGCTGGTGTGTAATTAC -3′) and Gli2 (5′- CCAACCAGAACAAGCAGAACA -3′) were cloned into the PLKO lentiviral vector. The PLKO construct with a scrambled shRNA sequence was used as a negative control. Lentiviral vector pSin4-EF2-IRES-Puro was used to generate expression constructs for tagged Gli, Jmjd3, Ash2L, WDR5 and EZH2. GliDBD fusion proteins were generated by fusing the Gli3 Zinc-finger domains (aa 477–636) with EZH2, Jmjd3 full-length protein or the C-terminal fragment including JmjC domain (aa 1,141–1,641). Lentiviruses were prepared according to a previously described procedure [12] . PolyJet (Signagen) was used for plasmid transfection of cultured cells. Attached cultured cells were infected at a multiplicity of infection (MOI) of 5 for 24 h in media with 8 μg ml −1 polybrene. RNA-seq Cultured primary MEFs (second passage) were treated with or without Shh-conditioned media for 24 h before harvesting. Total RNAs were extracted, and RNA-seq libraries were prepared using Illumina RNA-Seq Preparation Kit and sequenced by an HiSeq 2000 sequencer. RNA-seq reads were mapped using TopHat with default settings ( http://tophat.cbcb.umd.edu ). The mapped reads with the Phred quality score <20 were filtered out, whereas the duplicates were marked but not removed using SAMTOOLS [68] and PICARD ( http://picard.sourceforge.net ). Transcript assembly and transcript abundance quantification were carried out using CUFFLINKS, and then differential expression analysis between Shh-treated and untreated MEFs was performed using CUFFDIFF [69] The differentially expressed genes with P <0.05 were selected for histone modification analyses ( Supplementary Table 1 ). Immunoblotting For immunoblotting, cells or tissues were lysed in RIPA buffer (50 mM Tris, pH 8, 250 mM NaCl, 0.05% SDS, 0.5% DOC, 1% NP-40). Histone fractions were prepared with standard acid extraction (0.2 N HCl). Cell lysates or histone fractions were separated on SDS–PAGE (SDS–polyacrylamide gel electrophoresis) gels. Antibodies used were mouse monoclonal antibodies against Gli1 (#2643, Cell Signalling), HA (HA-7, Sigma), GAPDH (G9545, Sigma), H3K27me3 (#39536, Active Motif), H3H4me3 (ab8580, Abcam), H3K27Ac (ab4729, Abcam), histone H3 (ab1791, Abcam), Myc (9E10, Bishop), EZH2 (612667, BD Biosciences), SUZ12 (#3737, Cell Signalling) and FLAG (F1804, M2, Sigma). HRP-conjugated secondary antibodies were purchased from Jackson Immunology. Uncropped immunoblots are shown in Supplementary Fig. 17 . Immunohistology and in situ hybridization Timed mouse pregnancies were determined by plugging date as day 0.5. Haematoxylin and eosin (H&E) staining and immunostaining were performed on paraffin sections. Antibodies used were against Olig2 (AB9610, Chemicon), NKX2.2 (74.5A5-s, DSHB, University of Iowa), FoxA2 (4C7-s, DSHB, University of Iowa), EZH2 (#3737, BD Bioscience), H3K4me3 (C42D8, Cell Signaling) and H3K27me3 (07-449, Millipore). The images were visualized using an Olympus BX50 microscope. In situ hybridization analyses were performed as described previously [12] on cryosections (P5 cerebellum) or paraffin sections (E10.5 neural tubes). The Ptch1 and Jmjd3 probes correspond to nucleotides (nts) 850–1,637 and nts 925–1,720 of their cDNAs, respectively. Co-immunoprecipitation experiments Antibodies were against the HA-tag (ab9110, rabbit, Abcam) or FLAG-tag (F2426, M2 beads, Sigma). Shh-responsive NIH3T3 cells were transiently transfected with plasmids expressing HA- or FLAG-tagged proteins using PolyJet (Signagen). Mock transfection was used as the negative control. Cells were harvested 24–48 h after transfection and were lysed with co-IP Lysis Buffer (50 mM Tris, pH 8.0, 150 mM NaCl, 1 mM EDTA, 1% Triton X-100, with protease inhibitor freshly added). Cell lysates were snap-frozen in liquid nitrogen and then thawed on ice followed by sonication to facilitate cell lysis. After centrifugation, appropriate antibodies were added to pre-cleared cell lysate and incubated at 4 °C overnight. Samples were incubated with protein A beads (GE Healthcare) for 1 h; beads were washed with co-IP buffer four times. Precipitated proteins were eluted by boiling in 2 × Sample Buffer before SDS–PAGE and western blot analysis. For λ -phosphatase treatment, 400 U of enzyme (Sigma) was added to cell lysates followed by 30 min incubation at 37 °C. Chromatin immunoprecipitation ChIP experiments were performed as described previously [12] . Dissociated cells were crosslinked with PFA or double crosslinked with DSG (Pierce) and PFA, and sonicated to fragments (200–1,000 bp). Antibodies used were against H3K27me3 (07-449, Millipore), H3K4me3 (ab8580, Abcam), H3K27Ac (ab4729, Abcam), histone H3 (ab1791, Abcam), SUZ12 (#3737, Cell Signaling), EZH2 (612667, BD Bioscience), Jmjd3 (ab85392, Abcam) [70] , WDR5 (A302-429A, Bethyl Laboratories), HA (ab9110, Abcam) and FLAG (F1804, M2, Sigma). Rabbit IgG was used as a negative control. Precipitated DNA was purified and subjected to real-time PCR. RT–PCR and q-PCR RNAs from cells or tissues were extracted with TRIZOL (Invitrogen) or the RNeasy kit (Qiagen). cDNAs were synthesized by reverse transcription using Superscript III (Invitrogen), followed by PCR or quantitative PCR analysis. An ABI-7500 real-time PCR system was used for quantitative PCR. Levels of GAPDH mRNA were used to normalize input RNA. Graphics shown are representative of experiments performed in triplicate. Experiments were repeated for at least three times. Standard errors were calculated according to a previously described method [12] . The primer sequences are listed in the Supplementary Information . Statistical analysis Data are expressed as means±s.d. Statistical analysis was performed by either analysis of variance with ANOVA post hoc t -test for multiple comparisons or a two-tailed unpaired Student’s t -test. A P value of <0.05 was considered significant. How to cite this article: Shi, X. et al . An Epigenetic switch induced by Shh signalling regulates gene activation during development and medulloblastoma growth. Nat. Commun. 5:5425 doi: 10.1038/ncomms6425 (2014). Accession codes. NCBI SRA SRP047495 for RNA-seq analyses of Shh-responsive genes in MEF cells.